Misaligned sequencing reads from theGNAQ-pseudogene locus may yieldGNAQartefact variants 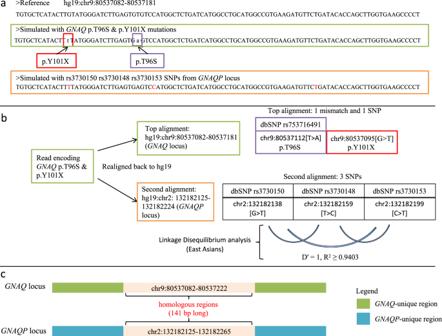Fig. 1: GNAQ p.T96S and p.Y101X mutations could be the results of misaligned sequencing reads from GNAQ-Pseudogene-1. aReference sequence fromGNAQlocus (top), in silico simulated read that would encode for GNAQ p.T96S and p.101X mutations (middle—green box) and in silico read that represents co-occurring SNPs, rs3730150, rs3730148 and rs3730153 (bottom—orange box; the co-occurring SNPs are in red).bTop-scoring alignments of the read that would encode for GNAQ p.T96S and p.101X. The read aligns to bothGNAQ(with one mismatch and one SNP) andGNAQP(with three SNPs) simultaneously. Linkage disequilibrium analysis of the three SNPs from theGNAQPlocus also showed that they tend to co-occur and cause an misalignment toGNAQlocus. This misalignment would yield the wrong callings of GNAQ p.T96S and p.101X mutations.cGNAQ-GNAQPhomologous regions that implicated p.T96S and p.Y101X, and rs3730150, rs3730148 and rs3730153 in theGNAQandGNAQPloci, respectively. The immediate regions outside of chr9:80537082-80537173 are unique toGNAQthat would further help Zhaoming Li et al. to further validate their current findings. Realignment of sequencing reads from GNAQ -pseudogene locus Genomic aligner BWA-MEM (v0.7.17-r1188) and reference genome hg19 were used to realign the sequencing data described in this study [2] . LDlink (version: March 2020) (public web tool: https://ldlink.nci.nih.gov/ ) was used to interrogate the prevalence of co-occurring polymorphisms that caused sequencing reads to misalign and produce the artefact calls reported by Zhaoming Li et al. Nature Communications 2019 [12] . Smith-Waterman alignment algorithm (version: March 2020) (public web tool: https://www.ebi.ac.uk/Tools/psa/emboss_water/ ) was used to derive the homologous GNAQ and GNAQP loci [13] .